Simultaneous enhancements in photon absorption and charge transport of bismuth vanadate photoanodes for solar water splitting n-Type bismuth vanadate has been identified as one of the most promising photoanodes for use in a water-splitting photoelectrochemical cell. The major limitation of BiVO 4 is its relatively wide bandgap ( ∼ 2.5 eV), which fundamentally limits its solar-to-hydrogen conversion efficiency. Here we show that annealing nanoporous bismuth vanadate electrodes at 350 °C under nitrogen flow can result in nitrogen doping and generation of oxygen vacancies. This gentle nitrogen treatment not only effectively reduces the bandgap by ∼ 0.2 eV but also increases the majority carrier density and mobility, enhancing electron–hole separation. The effect of nitrogen incorporation and oxygen vacancies on the electronic band structure and charge transport of bismuth vanadate are systematically elucidated by ab initio calculations. Owing to simultaneous enhancements in photon absorption and charge transport, the applied bias photon-to-current efficiency of nitrogen-treated BiVO 4 for solar water splitting exceeds 2%, a record for a single oxide photon absorber, to the best of our knowledge. The major challenge for solar hydrogen production is the reduction of hydrogen production cost comparable to that of fossil-based fuels [1] , [2] , [3] . To make solar hydrogen production a reality, a significant cost reduction for the construction of a photoelectrochemical cell (PEC) is critical [1] , [2] , [3] , [4] . Among various semiconductor electrodes (photoelectrodes) for use in PECs, oxide-based photoelectrodes have the possibility of significantly lowering the materials and processing costs while being stable in aqueous media [5] , [6] , [7] . n-Type bismuth vanadate (BiVO 4 ) has recently emerged as one of the most promising photoanodes for use in water-splitting PECs [8] , [9] , [10] , [11] . It absorbs a substantial portion of the visible spectrum (bandgap energy, ∼ 2.5 eV) and has a favourable conduction band edge position, which is very near the thermodynamic H 2 evolution potential [8] , [9] . As a result, it demonstrated the most negative photocurrent onset potential for water oxidation among all n-type semiconductors (photoanodes) having bandgaps in the visible region. Also, it appears to be fairly stable against chemical and photoelectrochemical corrosion [9] , [10] , [11] . A recent report shows that photoanodes composed of only oxide components, nanoporous BiVO 4 electrodes coupled with FeOOH and NiOOH as oxygen evolution catalysts [11] , can achieve an applied bias photon-to-current efficiency (ABPE) for water splitting as high as 1.7% in a stable manner (equation for ABPE is shown in Supplementary Information ) [12] . This result demonstrated the possibility for constructing a PEC for water splitting using only inexpensive and easy-to-process oxide components. One of the major limitations of BiVO 4 for further improving the solar energy conversion efficiency is its bandgap ( ∼ 2.5 eV), which fundamentally limits photon absorption. Considering that there are a substantial number of photons in the 2.0–2.5 eV region of the solar spectrum, a reduction in bandgap by even 0.1–0.3 eV can result in a significant efficiency increase [13] , [14] . For example, if a bandgap is reduced from 2.5 to 2.3 eV, the maximum photocurrent ( J max ) will increase from 6.47 to 9.12 mA cm –2 assuming 100% incident photon-to-current conversion efficiency (IPCE) for the photons that enable bandgap transition [13] . However, most previous doping studies of BiVO 4 were to increase carrier densities [15] , [16] , [17] , [18] . Studies reporting the change in photon absorption of BiVO 4 have been scarce and no clear elucidation of the effect of the dopants on the electronic band structures has been reported [19] , [20] . Considering that the valence band maximum (VBM) of BiVO 4 is significantly more positive than water oxidation potential, but the conduction band minimum (CBM) of BiVO 4 is very close to the reduction potential of water [8] , [9] , [21] , the reduction in bandgap of BiVO 4 will be the most advantageous if it is achieved by raising the VBM. In this study, we report that mild annealing treatment of nanoporous BiVO 4 under N 2 flow results in nitrogen incorporation into the oxygen sites, which effectively decreases the bandgap while also improving carrier mobility. In addition, we discover that the same N 2 treatment generates oxygen vacancies that can increase the majority carrier density. The effect of nitrogen incorporation and oxygen vacancies on the electronic band structure and charge transport of BiVO 4 are systematically elucidated by ab initio calculations, which corroborate well with the experimental results. Owing to concurrent enhancement in photon absorption, carrier density and carrier mobility, the N 2 -treated BiVO 4 electrode, when paired with oxygen evolution catalysts, breaks the wall of 2% ABPE for solar water splitting, a first for a single oxide photoelectrode. Synthesis and characterization Nanoporous BiVO 4 electrodes were first prepared by the method described in a recent study, which involves electrochemical deposition of BiOI followed by thermal and chemical conversion to BiVO 4 (ref. 11 ). Nitrogen doping of BiVO 4 was achieved by annealing the BiVO 4 electrodes at 350 °C for 2 h while flowing N 2 . This is an exceptionally gentle procedure for nitrogen doping considering that nitridation or nitrogen doping of oxides is generally achieved by annealing with a flow of NH 3 at much higher temperatures (≥500 °C) [22] , [23] , [24] , [25] . Annealing under N 2 flow may create oxygen deficiencies in oxide compounds but is usually considered insufficient for nitrogen doping. We believe that the nanoparticulate nature of the BiVO 4 electrodes played a role in enabling nitrogen doping under such mild conditions. The scanning electron microscopy images and X-ray diffraction studies of N 2 -treated BiVO 4 electrodes do not show noticeable changes from those of untreated BiVO 4 ( Fig. 1a–d ; Supplementary Fig. 1 ). The first indication of nitridation was observed when a drop of water was placed on the surface of these electrodes to compare their hydrophilicities ( Fig. 1e,f ). While the BiVO 4 sample showed a high affinity to water, as any oxide surface would, the N 2 -treated sample showed strong hydrophobicity, suggesting the possibility of nitridation, which can considerably change the hydrophilicity of the surface. 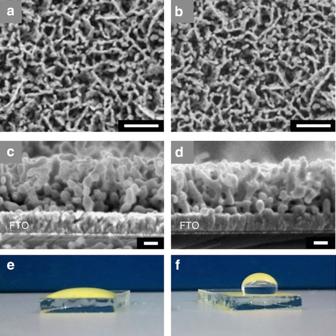Figure 1: SEM images and photographs. Top-view and side-view SEM images of (a,c) BiVO4and (b,d) N2-treated BiVO4. Photographs of a water droplet placed on (e) BiVO4electrode and (f) N2-treated BiVO4electrode. Scale bars, 1 μm for (a,b) and 200 nm for (c,d). Figure 1: SEM images and photographs. Top-view and side-view SEM images of ( a , c ) BiVO 4 and ( b , d ) N 2 -treated BiVO 4 . Photographs of a water droplet placed on ( e ) BiVO 4 electrode and ( f ) N 2 -treated BiVO 4 electrode. Scale bars, 1 μm for ( a , b ) and 200 nm for ( c , d ). Full size image The incorporation of nitrogen into the BiVO 4 lattice was confirmed by electron probe microanalyzer (EPMA) and X-ray photoelectron spectroscopy (XPS). For charge-balanced incorporation of nitrogen, three O 2− ions need to be removed for every two N 3− ions, creating one oxygen vacancy. Therefore, the formula of nitrogen-doped BiVO 4 can be written as BiVO 4−1.5 x N x if no other types of oxygen vacancies are present. The EPMA result showed that x is 0.31±0.05 (that is, BiVO 3.54 N 0.31 ). XPS study also confirmed the presence of nitrogen in the BiVO 4 lattice by showing a N 1 s peak ( Fig. 2a ) with the nitrogen content, x , estimated to be 0.34±0.02, which is comparable to the value obtained by EPMA. The location of the N 1 s peak (397–402 eV) agrees well with that of nitrogen incorporated into the oxide lattice [25] , [26] . The incorporation of N into the BiVO 4 lattice was further confirmed by Raman spectra that show significant broadening of various V–O stretching and VO 4 3− deformation modes of the bulk sample ( Supplementary Fig. 2 ) [27] , [28] . This indicates that unlike other oxides, nitrogen incorporation into BiVO 4 can occur using N 2 as the N source at mild temperatures. In fact, there exist two previous studies reporting nitrogen incorporation into vanadium oxides by annealing under N 2 flow [29] , [30] , suggesting relatively easy nitrogen incorporation into vanadium-based oxides. 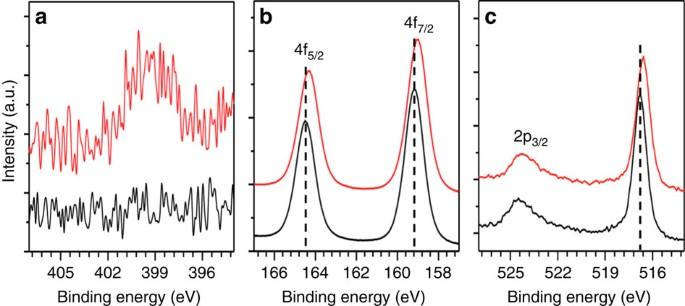Figure 2: XPS of BiVO4and N2-treated BiVO4. (a) 1speaks of N, (b) 4fpeaks of Bi and (c) 2ppeaks of V for BiVO4(black) and N2-treated BiVO4(red). Figure 2: XPS of BiVO 4 and N 2 -treated BiVO 4 . ( a ) 1 s peaks of N, ( b ) 4 f peaks of Bi and ( c ) 2 p peaks of V for BiVO 4 (black) and N 2 -treated BiVO 4 (red). Full size image The XPS study also revealed that the Bi 4 f and V 2 p peaks of N 2 -treated BiVO 4 were shifted to the lower binding energy ( Fig. 2b,c ). This should be due to the changes in local coordination environments of Bi and V ions, including a change in ligand type (O to N) and a decrease in coordination number due to oxygen vacancies compensating the charge difference between O 2− and N 3− . In addition, the possibility that the N 2 treatment created additional oxygen vacancies [31] , [32] , which would result in partial reduction of Bi 3+ and V 5+ ions, cannot be excluded. The ultraviolet–visible spectra of BiVO 4 and N 2 -treated BiVO 4 electrodes are shown in Fig. 3a . The N 2 -treated sample clearly showed a shift of the bandgap absorption to lower energy compared with untreated BiVO 4 . This agrees well with the darker yellow colour of the N 2 -treated BiVO 4 ( Fig. 3a , inset). The N 2 -treated BiVO 4 also shows a significant absorption before the absorption edge (wavelength >550 nm). This is most likely due to N 2 treatment generating significant disorder in the atomic arrangement (for example, O defects) on the surface of the high surface area nanoporous BiVO 4 electrode while incorporating nitrogen, creating interband states in the bandgap region [33] , [34] . The absorption due to these interband states makes it difficult to accurately assess the onset for the bandgap transition. 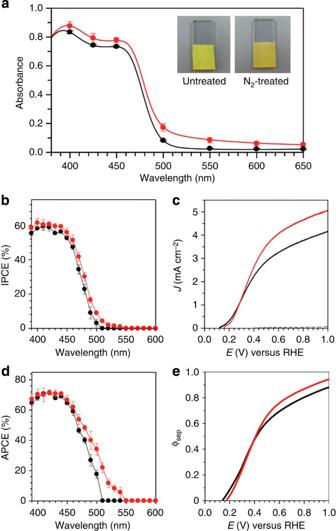Figure 3: Optical and photoelectrochemical properties. (a) Ultraviolet–visible absorption spectra with photographs of samples, (b) IPCE at 0.6 V versus RHE, (c)J–Vplots for sulfite oxidation under AM 1.5G, 100 mW cm–2illumination (scan rate, 10 mV s–1), (d) APCE at 0.6 V versus RHE and (e)φseps calculated from theJ–Vplots for BiVO4(black) and N2-treated BiVO4(red). A 0.5 M phosphate buffer (pH 7.2) containing 1 M Na2SO3was used as the electrolyte. The error bars were obtained by taking the s.d. values of measurements on three different samples. Figure 3: Optical and photoelectrochemical properties. ( a ) Ultraviolet–visible absorption spectra with photographs of samples, ( b ) IPCE at 0.6 V versus RHE, ( c ) J – V plots for sulfite oxidation under AM 1.5G, 100 mW cm –2 illumination (scan rate, 10 mV s –1 ), ( d ) APCE at 0.6 V versus RHE and ( e ) φ sep s calculated from the J – V plots for BiVO 4 (black) and N 2 -treated BiVO 4 (red). A 0.5 M phosphate buffer (pH 7.2) containing 1 M Na 2 SO 3 was used as the electrolyte. The error bars were obtained by taking the s.d. values of measurements on three different samples. Full size image Photo-oxidation of sulfite To determine the onset of photon absorption that contributes to the photocurrent generation, wavelength-dependent photocurrent was measured using monochromatic light for the photo-oxidation of sulfite and the IPCE was calculated. Since the oxidation kinetics of sulfite is fast, surface electron–hole recombination is negligible during photo-oxidation of sulfite. Therefore, photo-oxidation of sulfite enables a more precise estimation of photocurrent onset compared with photo-oxidation of water which typically suffers from slow oxidation kinetics and surface recombination. The IPCE result obtained at 0.6 V versus reversible hydrogen electrode (RHE) shows that the photocurrent onset of the N 2 -treated sample lies between 540 and 550 nm ( ∼ 2.27 eV) while that of the untreated sample lies between 500 and 510 nm ( ∼ 2.46 eV), which indicates a bandgap reduction of ∼ 0.2 eV for the N 2 -treated sample ( Fig. 3b ). The J – V plots of BiVO 4 and N 2 -treated BiVO 4 obtained using AM 1.5G illumination for sulfite oxidation are also shown in Fig. 3c . The N 2 -treated BiVO 4 electrode shows a significantly higher photocurrent than the BiVO 4 electrode. For example, the N 2 -treated sample generated a photocurrent density of 4.16±0.41 mA cm –2 at 0.6 V versus RHE while BiVO 4 generated 3.27±0.31 mA cm –2 at the same potential, corresponding to a 27% increase. This is the first example showing the generation of photocurrent higher than 4 mA cm –2 for any photo-oxidation reaction by any photoanode reported to date at a potential as low as 0.6 V versus RHE. If the photocurrent enhancement is due only to the enhanced photon absorption by the bandgap reduction, the N 2 -treated sample should show an increase in IPCE but not in the absorbed photon-to-current conversion efficiency (APCE). However, the N 2 -treated sample showed a considerable enhancement in APCE, particularly between 470 and 550 nm ( Fig. 3d ), indicating that the N 2 treatment also improved electron–hole separation. Indeed, the electron–hole separation yield, φ sep , of the N 2 -treated sample, which was calculated from the J – V plots obtained for sulfite oxidation, shows about an 8–10% increase at E >0.45 V versus RHE ( Fig. 3e ). For example, the electron–hole separation yields at 0.6 V versus RHE are 0.70±0.04 and 0.76±0.07 for untreated and N 2 -treated BiVO 4 , respectively. This means that the 27% photocurrent enhancement observed at 0.6 V for the N 2 -treated sample is partially due to an increase in photon absorption and partially due to an increase in electron–hole separation (see the Methods section and Supplementary Table 1 for detailed calculations). One plausible mechanism for N 2 treatment to increase φ sep is to increase the carrier density by creating extra oxygen vacancies, which can serve as donors, in addition to the oxygen vacancies created for charge-balanced substitution of N 3− with O 2− . This can result in an improvement in electron transport and, therefore, in electron–hole separation. The carrier densities in BiVO 4 and N 2 -treated BiVO 4 electrodes were compared by obtaining Mott–Schottky plots ( Supplementary Fig. 3 ). For nanoporous films, since the regions that contribute to space-charge layer capacitance and the corresponding surface area cannot be precisely quantified, accurate quantitative analysis of carrier density using Mott–Schottky analysis is not possible. However, since the samples compared in this study have exactly the same morphologies (particle sizes, aggregations and connectivities), relative qualitative comparison of carrier densities should be possible by comparing the magnitude of the slopes. The result shows that the slope of N 2 -treated BiVO 4 is ∼ 1/7 of the slope of BiVO 4 , indicating that the N 2 -treated BiVO 4 electrodes possess extra oxygen vacancies that serve as electron donors. This suggests that the record-high photocurrent shown in Fig. 3c is due to improved electron transport properties as well as bandgap reduction. An increase in n-type carrier density should result in a shift of flatband potential ( E FB ) to the negative direction. However, both the photocurrent onset and the E FB of the N 2 -treated sample are more positive than those of BiVO 4 ( Fig. 3c ; Supplementary Fig. 3 ). This is because the Helmholtz layer potential drop ( V H ) of the N 2 -treated BiVO 4 electrode, which is another factor that affects the position of E FB (ref. 35 ), is more positive than that of BiVO 4 , which is indicated by zeta potential measurements ( Supplementary Fig. 4 ). The change in V H of the N 2 -treated sample appears to cancel out the effect of an increased donor density on E FB . Density functional theory calculations The effect of charge-balanced N incorporation (that is, replacing three O 2− with two N 3− ) and of oxygen vacancies on the electronic band structure of BiVO 4 were studied using density functional theory (DFT) calculations, to gain insights into the changes occurring in BiVO 4 upon nitridation. Our experimental results show that in the N 2 -treated BiVO 4 , both N substitution and O vacancies are present at the same time, yielding a complex, combined effect on the electronic structure of BiVO 4 . Before investigating such combined effect, we discuss the electronic properties of N substitution and oxygen vacancies separately. We first performed spin-polarized calculations without addressing the charge imbalance between O 2− and N 3− . We used the Perdew–Burke–Ernzerh (PBE) [36] exchange correlation functional for pure BiVO 4 and BiVO 4 with 12.5% neutral O replaced with neutral N (1:1 substitution). We found that in the presence of N the bandgap of BiVO 4 was reduced by 0.5 eV ( Supplementary Fig. 5 ), mainly because of the hybridization of N and O 2 p states close to VBM. The presence of extra holes due to N substitution leads to two localized empty bands (level labelled ‘a’ in Supplementary Fig. 5b ) inside the bandgap of BiVO 4 . These bands will no longer be present when N substitution accompanies charge-balancing O vacancies, which will serve as electron donors and compensate for excess holes from N substitution, as discussed below (see also Supplementary Fig. 6 for the effect of artificially adding an electron per nitrogen to compensate for the excess holes from N substitution). To understand the effect of O vacancies separately, we performed spin-polarized calculations at two different vacancy concentrations of 6 and 1.5%, using PBE and PBE with Hubbard U -corrections [37] (PBE+ U , effective U (V)=2.7 eV) [17] , to verify the robustness of our results with respect to the functional adopted in our calculations. Both at the PBE and PBE+ U levels of theory, at the two concentrations, we found that the presence of O vacancies, which were created by removing neutral O atoms, did not lead to any modification of the bandgap of BiVO 4 (for details see Supplementary Figs 7 and 8 ). We also observed the formation of localized, filled states inside the bandgap of pristine BiVO 4 . Interestingly, the spin density of the gap states is localized on V, as shown in Supplementary Fig. 8 , causing local lattice distortions (in addition to those induced by missing O atoms), and indicating the formation of small polarons. Indeed, small polarons are likely to form in oxides such as BiVO 4 that exhibit strong electron–phonon interaction, as indicated, for example, by the large difference between the high frequency and static dielectric constants ɛ (the high frequency and static ɛ , averaged over the three lattice directions, are 6.9 and 52, respectively, as computed by density functional perturbation theory [38] for pure BiVO 4 ). Our results on the formation of small polarons are consistent with recent mobility measurements on single crystal n -type BiVO 4 , which reported very low electron mobilities [39] ( ∼ 0.2 cm –2 V –2 s –1 ) and suggested that the conduction of electrons is dominated by small polaron hopping. Previous calculations showed that O vacancies lead to shallow donor levels in BiVO 4 (ref. 31 ), with negative ionization energies for E (V 0 /V 2+ ) and that the only stable charged state for an O vacancy in BiVO 4 is q =+2 due to the spontaneous ionization of two electrons, regardless of the Fermi level position [40] . These results are consistent with our finding that the two electrons present at an O vacancy site are ionized and localized at V atoms, thus forming small polarons. Similar findings for SrTiO 3 have also been discussed in a recent study by Janotti et al . [41] We also computed the small polaron binding energy [42] , that is, the energy difference between bound small polarons and free carriers. We found a non-negligible value of ∼ 0.50 eV indicating that the formation of small polarons is energetically favourable (see Methods for calculation details). Having established the separate effects of N substitution and O vacancies on the electronic structure of BiVO 4 , we now turn to analyze their combined effect. In the case of charge-balanced N substitution (9% O replaced with 6% N and 3% O vacancy) we found that no states are formed in the bandgap of BiVO 4 , as shown in Fig. 4a . This is because the electrons ionized from O vacancies compensate for the holes generated by N substitution, thus balancing the charge. No small polaron is formed at the vanadium sites in this case. The important finding is that the bandgap is still lowered by 0.3–0.4 eV (depending on the location in the lattice of the substituted N) compared to that of pure BiVO 4 . The computed projected density of states (as shown in Supplementary Fig. 9 ) showed that the VBM has contributions from both O and N 2p states, similar to the case of N substitution discussed earlier. With lower doping concentration (4.5% O replaced with 3% N and 1.5% O vacancy), the VBM moves upward by 0.2 eV compared with that of pure BiVO 4 . In sum, we found that in the presence of N substitution and charge-compensating O vacancies, the bandgap decrease is similar to that obtained in the case where only substitutional N is present, and the bandgap decrease is more pronounced with increasing N concentration. 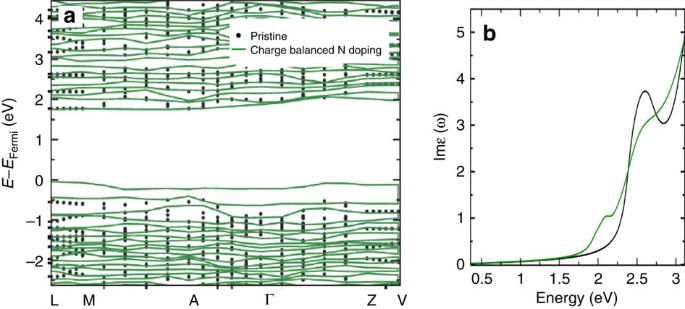Figure 4: Comparison of pristine and charge-balanced N-doped BiVO4. (a) Band structures and (b) simulated absorption spectra (imaginary part of dielectric function) of pristine BiVO4(black) and BiVO4with charge-balanced N-doping (9% O replaced with 6% N and 3% O vacancy) (green). An artificial broadening 0.08 eV is applied to take into account the finite temperature and phonon effects. The highest occupied level at 0 K of BiVO4with charge-balanced N-doping was taken as the Fermi level (EFermi). Figure 4: Comparison of pristine and charge-balanced N-doped BiVO 4 . ( a ) Band structures and ( b ) simulated absorption spectra (imaginary part of dielectric function) of pristine BiVO 4 (black) and BiVO 4 with charge-balanced N-doping (9% O replaced with 6% N and 3% O vacancy) (green). An artificial broadening 0.08 eV is applied to take into account the finite temperature and phonon effects. The highest occupied level at 0 K of BiVO 4 with charge-balanced N-doping was taken as the Fermi level ( E Fermi ). Full size image The information on energy levels provided by band structure calculations is insufficient to investigate light absorption efficiency of BiVO 4 . Hence, we also computed the optical transition probabilities from valence to conduction states for pristine and charge-balanced N-doped BiVO 4 (9% O replaced with 6% N and 3% O vacancy) and simulated absorption spectra using the random phase approximation including local field effects [43] . Although this approximation neglects excitonic effects, we expect it to be accurate to account for changes in absorption spectra when N is added to the sample [44] . We estimated the change of the exciton binding energy before and after doping by using a hydrogen-like model and we found it is of the order of 0.05 eV (see Methods for details). The spectra were averaged over three lattice directions to compare with experimental results obtained from polycrystalline samples. The resulting simulated absorption spectra show that the absorption edge of N-doped BiVO 4 is lower than that of the pristine BiVO 4 by about 0.3 eV ( Fig. 4b ), confirming that charge-balanced N substitution can indeed enhance visible light absorption at lower energy. This result agrees well with our experimental observation that incorporating ∼ 8% N results in a 0.2 eV reduction of the bandgap. Our experimental results suggest that in addition to the O vacancies caused by charge-balanced replacement of O 2− with N 3− , additional oxygen vacancies are present serving as electron donors in N 2 -treated BiVO 4 . Therefore, we performed calculations of N-doped BiVO 4 with excess O vacancies (6% N and 6% O vacancy) ( Fig. 5 ; Supplementary Fig. 10 ), where half of the O vacancies balance the charges of substitutional N atoms, and the other half provide extra electrons to form polarons. We observed both a reduction of the bandgap by 0.3 eV ( Fig. 5a ), compared with that of pristine BiVO 4 , and the formation of small polarons localized on V atoms ( Fig. 5b ). 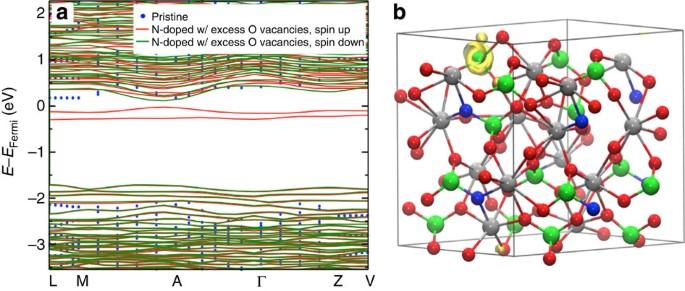Figure 5: Calculation results for N-doped BiVO4with excess O vacancies. (a) Comparison of band structures of pristine BiVO4(blue dot) and N-doped BiVO4with excess O vacancies (6% N and 6% O vacancy) with spin up (red) and spin down (green) configurations. The highest occupied level at 0 K of N-doped BiVO4with excess O vacancies (spin up configuration) was taken as the Fermi level (EFermi). (b) Spin density map of N-doped BiVO4with excess O vacancies showing the localization of an electron on V. The spin density isosurface (0.0049, e bohr−3) of an isolated band (around the Fermi level at theΓpoint) is shown in yellow; atoms are represented by spheres: V (green), Bi (silver), O (red) and N (blue). Projected density of states is shown inSupplementary Fig. 10. Figure 5: Calculation results for N-doped BiVO 4 with excess O vacancies. ( a ) Comparison of band structures of pristine BiVO 4 (blue dot) and N-doped BiVO 4 with excess O vacancies (6% N and 6% O vacancy) with spin up (red) and spin down (green) configurations. The highest occupied level at 0 K of N-doped BiVO 4 with excess O vacancies (spin up configuration) was taken as the Fermi level ( E Fermi ). ( b ) Spin density map of N-doped BiVO 4 with excess O vacancies showing the localization of an electron on V. The spin density isosurface (0.0049, e bohr −3 ) of an isolated band (around the Fermi level at the Γ point) is shown in yellow; atoms are represented by spheres: V (green), Bi (silver), O (red) and N (blue). Projected density of states is shown in Supplementary Fig. 10 . Full size image We also note that N-doping increases the mobility of small polarons by changing the static dielectric constant of BiVO 4 (ref. 45 ). Our computation shows that small polarons’ activation energy of N-doped BiVO 4 (6% N substitution and 3% O vacancies) is lowered by 1.1% and, as a result, the electron mobility is increased by 25% according to the small polaron model (see the Methods section for the computation details) [39] , [42] . This means that the measured, enhanced φ sep of the N 2 -treated sample is not only due to an increase in carrier density but also due to an increase in carrier mobility. To confirm this, we prepared H 2 -treated BiVO 4 that has the same O vacancy concentration and, therefore, the same carrier density as the N 2 -treated sample but no N incorporation ( Supplementary Fig. 11 ) [31] . By comparing electron transport properties of the two samples using APCEs and photocurrents generated by front-side and back-side illuminations ( Supplementary Figs 11 and 12 ) [16] , [46] , [47] , [48] , we observed that the electron transport of N 2 -treated samples is more enhanced than that of H 2 -treated samples. This result suggests that other than the carrier density increase by O vacancies that are common for H 2 -treated and N 2 -treated samples, the N 2 -treated samples have an additional factor improving electron transport. This agrees well with the result from the polaron activation energy calculation that N incorporation results in an increase in polaron mobility. Altogether, our experimental and computational results show that the simple and mild N 2 treatment used in this study simultaneously enhanced photon absorption, carrier density and carrier mobility, all of which are critical for improving the photoelectrochemical properties of BiVO 4 . Photo-oxidation of water The ability of N 2 -treated BiVO 4 electrode to photoelectrolyze water was examined in a 0.5 M phosphate buffer (pH 7.2) after oxygen evolution catalysts (OECs), FeOOH and NiOOH, were photodeposited on the N 2 -treated BiVO 4 surface sequentially; a FeOOH layer was first photodeposited on the N 2 -treated BiVO 4 surface followed by the deposition of a NiOOH (see Methods for the synthesis details). It was reported that the BiVO 4 /FeOOH interface minimizes electron–hole recombination at the BiVO 4 /FeOOH junction and the NiOOH/electrolyte surface makes the surface charge more favourable while concurrently improving the water oxidation kinetics [11] . As a result, the dual catalyst layer structure provided the best performance compared with single layer or the OEC layers with the reversed order. Since the surface of the N 2 -treated BiVO 4 electrode is expected to be quite different from that of the untreated BiVO 4 electrode (for example, surface charge and surface termination), the N 2 -treated BiVO 4 /FeOOH interface may no longer be ideal. However, depositing the same OECs on BiVO 4 and N 2 -treated BiVO 4 would allow us to examine any changes at the BiVO 4 /OEC junction and for solar water oxidation caused solely by N 2 treatment. The results show that N 2 treatment increased the photocurrent density for water oxidation at 0.6 V versus RHE from 2.71 to 3.47 mA cm –2 ( Fig. 6a ). The J – V curve was also measured using a two-electrode cell to calculate ABPE ( Fig. 6b ). The highest ABPE, 2.2%, was achieved at 0.58 V, which is the record-high ABPE attained by a single oxide photon absorber to date ( Fig. 6c ). The Faradaic efficiency for O 2 evolution at 0.6 V versus RHE was 96% ( Fig. 6d ). The ratio of H 2 :O 2 produced was 1.81:1 ( Fig. 6d ). Considering that there are no competing reactions available at the cathode, the slight deviation from the stoichiometric H 2 /O 2 production is due to the leak of H 2 during manual sampling of H 2 for gas chromatography analysis. 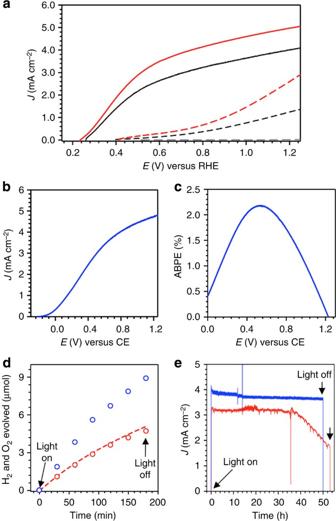Figure 6: Photoelectrochemical water-splitting performance. (a)J–Vplots of BiVO4/FeOOH/NiOOH (black, solid), N2-treated BiVO4/FeOOH/NiOOH (red, solid), BiVO4(black, dashed), and N2-treated BiVO4(red, dashed) measured in a 0.5 M phosphate buffer (pH 7.2) under AM 1.5G illumination using a three-electrode cell. Grey dashed lines show dark current of N2-treated BiVO4/FeOOH/NiOOH. (b)J–Vplot and (c) ABPE of N2-treated BiVO4/FeOOH/NiOOH obtained using a two-electrode cell for solar water splitting (CE: counter electrode). (d) Detection of H2(blue) and O2(red) produced by N2-treated BiVO4/FeOOH/NiOOH at 0.6 V versus counter electrode. The red dashed line represents the amount of O2calculated assuming 100% Faradaic efficiency. (e)J–tplots of N2-treated BiVO4for sulfite oxidation (blue) and N2-treated BiVO4/FeOOH/NiOOH for water oxidation (red) at 0.6 V versus RHE. Figure 6: Photoelectrochemical water-splitting performance. ( a ) J – V plots of BiVO 4 /FeOOH/NiOOH (black, solid), N 2 -treated BiVO 4 /FeOOH/NiOOH (red, solid), BiVO 4 (black, dashed), and N 2 -treated BiVO 4 (red, dashed) measured in a 0.5 M phosphate buffer (pH 7.2) under AM 1.5G illumination using a three-electrode cell. Grey dashed lines show dark current of N 2 -treated BiVO 4 /FeOOH/NiOOH. ( b ) J–V plot and ( c ) ABPE of N 2 -treated BiVO 4 /FeOOH/NiOOH obtained using a two-electrode cell for solar water splitting (CE: counter electrode). ( d ) Detection of H 2 (blue) and O 2 (red) produced by N 2 -treated BiVO 4 /FeOOH/NiOOH at 0.6 V versus counter electrode. The red dashed line represents the amount of O 2 calculated assuming 100% Faradaic efficiency. ( e ) J–t plots of N 2 -treated BiVO 4 for sulfite oxidation (blue) and N 2 -treated BiVO 4 /FeOOH/NiOOH for water oxidation (red) at 0.6 V versus RHE. Full size image The long-term stability of N 2 -treated BiVO 4/ FeOOH/NiOOH for water oxidation was examined by measuring J–t plots at 0.6 V versus RHE and was compared with the long-term stability of N 2 -treated BiVO 4 for sulfite oxidation at the same potential ( Fig. 6e ). The photocurrent for sulfite oxidation was stable for 50 h and no sign of decay was observed, suggesting that the presence of nitrogen and oxygen vacancies in the lattice are stable under illumination and electrical bias. The photocurrent for water oxidation was stable for 30 h but after 30 h it gradually decreased. Considering the photostability of N 2 -treated BiVO 4 for sulfite oxidation and the previously reported photostability of undoped BiVO 4 combined with the same OECs for water oxidation [11] , the instability observed during photo-oxidation of water is most likely due to the instability of the N 2 -treated BiVO 4 /OEC junction resulting in the loss of OECs over time, which was confirmed by XPS studies ( Supplementary Fig. 13 ). These results suggest that while N 2 -treated BiVO 4 itself is compositionally stable, it will require new OECs to form a more stable N 2 -treated BiVO 4 /OEC interface to achieve a long-term stability for photo-oxidation of water. Annealing of nanoporous BiVO 4 at 350 °C under N 2 flow resulted in substitutional incorporation of nitrogen and the formation of O vacancies, which simultaneously enhanced photon absorption, carrier density and carrier mobility. The effect of N incorporation and O vacancies in the BiVO 4 lattice were thoroughly examined experimentally and computationally to provide new understanding of the electronic band structures and photoelectrochemical properties of BiVO 4 . Charge-balanced N-doping (that is, 9% O replaced with 6% N and 3% O vacancy) reduced the bandgap of BiVO 4 by elevating the VBM without introducing mid-gap states in the bandgap region. N-doping also decreased the static dielectric constant of BiVO 4 and improved the mobility of electrons, which are small polarons. In addition to the O vacancies required for charge-balanced N-doping, the N 2 -treated BiVO 4 contained additional oxygen vacancies, which served as electron donors in N 2 -treated BiVO 4 . As a result, the major carrier density as well as the major carrier mobility of BiVO 4 could be increased by the simple N 2 treatment. The experimental and theoretical studies reported herein may serve as guidelines to further improve photon absorption and charge transport of BiVO 4 -based photoanodes for more practical and efficient solar water splitting. For example, predicting and incorporating a dopant that can simultaneously improve photon absorption and charge transport may serve as an effective strategy to improve photoelectrochemical performance. Future studies should also include identifying OECs that can optimally interface with BiVO 4 electrodes with modified compositions. Nitrogen incorporation into BiVO 4 The nanoporous BiVO 4 electrode used in this study was prepared using the same method reported in our recent paper [11] , [49] . Nitrogen incorporation was achieved by annealing the BiVO 4 electrodes at 350 °C for 2 h in a tube furnace while flowing N 2 . This annealing condition was identified as optimal to generate samples with the best photoelectrochemical properties after trying various annealing temperatures (300–450 °C, ramping rate=5 °C min –1 ) and annealing times (1–3 h). The N incorporation shown in this study is the maximum N incorporation that can be achieved by N 2 treatment. Increasing temperature or duration of N 2 treatment did not increase the N incorporation. When the duration of N 2 treatment is shortened, the amount of N incorporated could be reduced but the photocurrent enhancement was also reduced. For example, when the annealing time at 350 °C while flowing N 2 was reduced from 2 h to 30 min, the N content, x , in BiVO 4−1.5 x N x was reduced from=0.33 to 0.10 judging from the XPS results and the photocurrent density at 0.6 V versus RHE was reduced from 4.2 to 3.4 mA cm –2 . Photodeposition of FeOOH/NiOOH OECs on N 2 -treated BiVO 4 electrodes The photodeposition of dual-layer oxygen evolution reaction catalysts (that is, FeOOH and NiOOH) on the surface of the N 2 -treated BiVO 4 photoanode were performed using the method described in our recent paper [11] with a few modifications. Before photodeposition, the N 2 -treated BiVO 4 was first immersed in 1 M NaOH solution for ∼ 1–2 min to ensure the wetting of its hydrophobic surface. After rinsing the surface with DI water, the photodeposition of FeOOH was carried out in a 0.1 M FeSO 4 solution (pH 3.2–3.8) while gently stirring. Before photodeposition, the solution was purged with nitrogen gas for 1 h. An undivided three-electrode cell composed of a N 2 -treated BiVO 4 working electrode, a Pt counter electrode, and a Ag/AgCl (4 M KCl) reference electrode, was used. A 300 W Xe arc lamp (Oriel Newport) with an AM 1.5G filter, neutral density filters and a water filter (IR filter) was used as the light source. The light was illuminated through the FTO contact (back-side illumination) and the light intensity at the FTO surface was adjusted to be 1 mW cm –2 using a research radiometer (International Light, IL 1700) coupled with a thermopile detector (International Light, SED623/H/N/K15). To facilitate photodeposition, an external bias of ca. 0.26–0.31 V versus Ag/AgCl (4 M KCl), which was the open circuit potential of the N 2 -treated BiVO 4 electrodes in the solution in dark, was applied using a potentiostat (BioLogic SP-200). After the photodeposition of FeOOH, the electrodes were rinsed with DI water and dried at room temperature. Among various photodeposition times tested (that is, 10–60 min), deposition for ca. 45 min (passing a total charge of 65–70 mC cm –2 ) was identified to be optimum to maximize photocurrent generation for water oxidation. Photodeposition of NiOOH was carried out on the N 2 -treated BiVO 4 /FeOOH electrodes using a 0.1 M NiSO 4 solution with pH adjusted to 6.3–7.0 by adding NaOH. To facilitate photodeposition, an external bias of ca. 0.12–0.16 V versus Ag/AgCl (4 M KCl), which was the open circuit potential of the N 2 -treated BiVO 4 /FeOOH electrodes in the solution in dark, was applied. The optimum deposition time was ca. 25 min (passing a total charge of 20–22 mC cm –2 ). After photodeposition of NiOOH, NiOOH was also electrochemically deposited by applying +1.2 V versus Ag/AgCl (4 M KCl) for 1 min. This was to deposit NiOOH on any bare BiVO 4 or FTO surfaces exposed to the electrolyte. After deposition, the electrodes were washed with DI water and dried at room temperature. The molar ratio of Fe/Ni in optimized N 2 -treated BiVO 4 /FeOOH/NiOOH electrodes was estimated to be 4.92±1.87 by energy-dispersive spectroscopy (using three samples at the 95% confidence level). Characterization The purity and crystal structure of the synthesized electrodes, pristine BiVO 4 and N 2 -treated BiVO 4 , were examined by X-ray diffraction (Bruker D8 Advanced PXRD, λ =1.5418 Å, 298 K, Ni-filtered Cu K α -radiation). The crystal morphologies of the electrodes were examined with scanning electron microscopy using a LEO 1530 microscope at an accelerating voltage of 5 kV. The chemical composition of Bi/V in the BiVO 4 electrodes was confirmed to be 0.98±0.02 by a Hitachi S3400-N microscope equipped with an energy-dispersive X-ray spectrometer (Thermo Fisher Scientific Inc.). For the quantitative analysis of the amount of nitrogen doping in N 2 -treated BiVO 4 , EPMA employing a CAMECA SX-50 apparatus was conducted. In sample preparation, the anode material on the FTO film was scraped off and placed on a carbon tape. A precisely quantitative analysis of nitrogen was achieved by calibration using a high-purity GaN as a standard reference. Ultraviolet–visible absorption spectra were obtained on a Cary 5000 Ultraviolet–visible spectrophotometer (Agilent), in which the sample electrode was fixed in the centre of an integrating sphere to measure all light reflected and transmitted to accurately assess the absorbance. FTO glass was used as the reference for these absorption measurements. XPS spectra were recorded using a K-Alpha X-ray photoelectron spectrometer (Thermo Scientific Inc.) equipped with a monochromated Al K α line as the X-ray source. The binding energies were calibrated with respect to the residual C (1 s ) peak at 284.6 eV. Raman spectra of the pristine BiVO 4 and the N 2 -treated BiVO 4 electrodes were recorded at room temperature using a Raman spectrometer (Thermo Scientific DXR smart Raman spectrometer). A red laser (780 nm) was used as excitation source. The electrodes were placed such that the BiVO 4 and the N 2 -treated BiVO 4 side of electrodes faced the laser source. Capacitance measurements for Mott–Schottky plots were obtained using a SP-200 potentiostat/EIS (BioLogic Science Instrument) with an EC-Lab software package. A sinusoidal modulation of 10 mV was applied at frequencies of 0.5 and 1 kHz. The three-electrode setup was used in a 0.5 M phosphate buffer solution (pH 7.2). All electrodes were masked with epoxy resin to expose the same geometrical area (ca. 0.1 cm 2 ) for this measurement. The zeta potential measurements of pristine BiVO 4 and N 2 -treated BiVO 4 were conducted using a zeta potential analyser (Micromeritics NanoPlus-2), which measures electrophoretic mobilities of charged particles to calculate zeta potentials. This was to compare Helmholtz layer potential drop ( V H ) of the pristine and N 2 -treated BiVO 4 electrodes (equation 1), which is another factor that affects the position of flatband potential ( E FB ) (equation 2) [35] . The point of zero zeta potential (pH PZZP ) of BiVO 4 and N 2 -treated BiVO 4 could not be directly measured because BiVO 4 is not chemically stable near its pH PZZP. However, zeta potentials at pH 7.2 solution could still be used to qualitatively compare the pH PZZP s of BiVO 4 and N 2 -treated BiVO 4 and their effects on E FB . For the zeta potential measurement, BiVO 4 and N 2 -treated BiVO 4 nanoparticles were scratched off the electrode substrates and dispersed in a 0.5 M phosphate buffer solution (pH 7.2) using sonication. Photoelectrochemical measurements Photoelectrochemical performances of photoanodes prepared in this work were evaluated in a typical undivided three-electrode configuration using a SP-200 potentiostat/EIS (BioLogic Science Instrument). The simulated solar illumination was obtained by passing light from a 300 W Xe arc lamp (Oriel Newport) through a water filter (IR filter)/neutral density filters/an AM 1.5G filter. Illumination through the FTO side (back-side illumination) was used. The power density of the incident light was calibrated to 100 mW cm –2 at the surface of the FTO substrate (before the light penetrates FTO) by using a research radiometer (International Light, IL 1700) coupled with a thermopile detector (International Light, SED623/H/N/K15) and a NREL certified reference cell (Photo Emission Tech., Inc.). The beam passed through an optical fibre and the active area of the sample exposed to electrolyte is between ca. 0.1–0.2 cm 2 . Photocurrent measurements were performed in a 0.5 M potassium phosphate (KH 2 PO 4 ) buffer solution (pH 7.2) with or without 1 M sodium sulfite (Na 2 SO 3 ) as a hole scavenger. Before measurements, the electrolyte was thoroughly deaerated by purging with nitrogen. Photocurrents were monitored either while sweeping the potential to the positive direction with a scan rate of 10 mV s −1 or while applying a constant bias. The mean values and confidence intervals of photocurrent density and electron–hole separation yield provided in the text and Supplementary Table 1 were determined using measurements on three different samples at the 95% confidence level. While all measurements were carried out using a Ag/AgCl (4 M KCl) reference electrode, all results in this work were presented against the RHE for ease of comparison with H 2 and O 2 redox levels and other reports that used electrolytes with different pH conditions. The conversion between potentials versus Ag/AgCl and versus RHE is determined using the equation below. IPCE at each wavelength was determined using illumination from a 300 W Xe arc lamp (Oriel Newport) passed through an AM 1.5G filter, neutral density filters, and a water filter to approximate the output of the sun. Monochromatic light was produced using an Oriel Cornerstone 130 monochromator with a 10-nm bandpass. The intensity of incident light was measured using a research radiometer (International Light, IL 1700) with a calibrated silicon photodiode detector (International Light, SED033). IPCE was measured in 0.5 M phosphate buffer (pH 7.2) with the same three-electrode setup described above for photocurrent measurements, using a Princeton Applied Research Potentiostat/Galvanostat model 263A to apply 0.6 V versus RHE. APCE was obtained by dividing the IPCE by the light harvesting efficiency at each wavelength using the following equations (equations 4 and 5). To calculate respective J max s (maximum photocurrent density achievable assuming 100% IPCE for photons with energy ≥ E g ) of BiVO 4 and N 2 -treated BiVO 4 , the National Renewable Energy Laboratory (NREL) reference solar spectral irradiance at AM 1.5G (radiation energy (W m −2 nm −1 ) versus wavelength (nm)) was first converted to the solar energy spectrum in terms of number of photons (s −1 m −2 nm −1 ) versus wavelength (nm) [50] . Then, the number of photons above the bandgap energy of each sample shown in this study was calculated using a trapezoidal integration (in 10 nm increments) of the spectrum and was converted to the current density (mA cm −2 ). J max s for pristine BiVO 4 and N 2 -treated BiVO 4 were 6.47 and 9.12 mA cm –2 , respectively. To calculate J abs (photocurrent assuming 100% APCE), the light harvesting efficiency at each wavelength was multiplied during each step of the trapezoidal integration. Using these calculations, J abs s for pristine BiVO 4 and N 2 -treated BiVO 4 were calculated to be 4.44±0.05 mA cm –2 and 5.30±0.07 mA cm –2 , respectively. Photocurrent density obtained for sulfite oxidation was used to calculate the electron–hole separation yield (=the yield of the photogenerated holes that reach the surface), φ sep , using the following equation (equation 6), where J PEC is the measured photocurrent density and φ ox is the yield of the surface reaching holes that are injected into the solution species [51] , [52] . For sulfite oxidation with extremely fast oxidation kinetics, surface recombination is negligible and φ ox is ∼ 1. Therefore, φ sep is obtained by dividing J PEC by J abs . The ABPE was calculated from the J–V curves obtained from a two-electrode systems assuming 100% Faradaic efficiency using the following equation, where J is the photocurrent density, V bias is the applied bias between working electrode (BiVO 4 photoanode) and counter electrode (Pt cathode) and P in is the incident illumination power density (AM 1.5G, 100 mW cm –2 ) (equation 7) [12] . O 2 measurements were performed using an Ocean Optics fluorescence-based oxygen sensor (Neofox, FOSPOR-R 1/16″). The probe measures the O 2 content in the headspace as mole%, which was converted to micromoles after adjusting for the O 2 dissolved in solution using Henry’s Law. O 2 measurements were performed with an undivided two-electrode cell using a custom built and airtight 3-neck 50 ml round-bottom flask with a N 2 -treated BiVO 4 /FeOOH/NiOOH working electrode and a Pt mesh counter electrode. O 2 measurements were carried out while applying 0.6 V between the working electrode and the counter electrode. The experiment of oxygen evolution was run for 3 h after a 15-min waiting period at open circuit. The 15 min periods before and after the oxygen evolution step were used to calculate the O 2 leak rate of the cell. The amount of O 2 detected was divided by the amount of O 2 expected calculated from photocurrent assuming 100% Faradaic efficiency to calculate the true Faradaic efficiency or the photocurrent-to-O 2 conversion efficiency. H 2 production measurements were carried out by applying 0.6 V between the working electrode and the counter electrode (two-electrode system) under the same condition used in O 2 measurement, using GC (SRI Instruments) to analyze the headspace. The amount of H 2 gas evolved was determined by taking 100 μl of gas from the headspace of the cell using a syringe and injecting it into the gas-sampling loop of the GC every one hour. The GC was equipped with a packed MolSieve 13 X column. Helium (Airgas, ultra high purity) was used as the carrier gas. A helium ionization detector was used to quantify hydrogen concentration. All the confidence intervals for any quantity shown in the main text were calculated using the 95% confidence level. DFT calculations for nitrogen substitutions Calculations were performed with the Quantum Espresso Package [53] using DFT with the generalized gradient approximation and the parameterization proposed by PBE [36] . We used ultrasoft pseudo-potentials, where (3 s , 3 p ) electrons of V were included in the valence partition. A kinetic energy cutoff of 40 and 240 Ry for the wavefunction and charge density, respectively, and (4 × 3 × 6) Monkhorst–Pack k-point grids were used in geometry optimizations, and (5 × 5 × 7) k-point grids were used for density of states calculations. In our super cell calculations, both internal geometry and cell size were fully optimized for pristine BiVO 4 and only the internal geometry was optimized for N-doped BiVO 4 . We obtained a bandgap of 2.25 eV for pristine BiVO 4 , underestimating the experimental optical gap by only ∼ 0.2 eV. The good agreement between the computed bandgap and the experimental optical gap is due to a partial cancelation of errors, encompassing the PBE underestimation of gaps, the neglect of excitonic effects (the exciton binding energy is estimated to be ∼ 0.23 eV) and spin-orbit coupling ( ∼ 40 meV, as obtained by fully relativistic calculations). The exciton binding energy was estimated using a hydrogen-like model, ( E b : the binding energy of the first excitonic state; m: the effective mass, ; ɛ ∞ : the high-frequency dielectric constant). Our results for the band structure of the N-doped oxide (12.5% O atoms replaced with N, equivalent to the stoichiometry BiVO 3.5 N 0.5 ) are shown in Supplementary Fig. 5 for the spin-polarized configuration, which was found to be energetically favoured. The 1:1 substitution of O with N cannot compensate for the charge change caused by the loss of an O atom. (Oxygen has 6 valence electrons and N has 5 valence electrons.) The resulting presence of excess holes leads to two localized empty bands (labelled ‘a’ in Supplementary Fig. 5b ) inside the bandgap of BiVO 4 . The energy of the localized mid-gap states is sensitive to the location of N atoms in the lattice (it varies by 0.5 eV depending on the position of the N atom). The bandgap of N-doped BiVO 4 , defined as the energy difference between the top of the valence band (level labelled ‘b’ in Supplementary Fig. 5b ) and the bottom of the conduction band (level labelled ‘c’ in Supplementary Fig. 5b ), is 1.77 eV at 12.5% N-doping, i.e. 0.48 eV lower than that of pristine BiVO 4 . These bands are no longer present in the case of N substitution accompanied by charge-balancing O vacancies, which will serve as electron donors and compensate for the excess holes present due to N substitution ( Fig. 4a ). We also show the band structure of the N-doped oxide (12.5% O replaced with N) when we artificially added an electron per nitrogen to compensate for excess holes generated from charge-imbalanced N substitution ( Supplementary Fig. 6 ). (In other words, we artificially substituted O with N − ). Our results show that the bandgap of N doped BiVO 4 is 1.86 eV at 12.5% N-doping, that is, 0.39 eV lower than that of pristine BiVO 4 . However, in this case the mid-gap states are no longer present. The projected density of states in Supplementary Fig. 6a shows that there is significant hybridization between N 2 p and O 2 p states at the top of the valence band. DFT calculations for oxygen vacancies Calculations were performed using spin-polarized DFT and the PBE approximation. We also included Hubbard U -corrections to the d electrons of V ( U =2.7 eV) following a previous study by Park et al . [17] . All O vacancies discussed in this study were created by removing neutral O atoms. At the PBE level of theory, when 1.5 or 6% O vacancies were introduced in the system, we observed the appearance of one isolated band inside the bandgap of BiVO 4 (shown in Supplementary Fig. 7 ), whose bandgap and insulating character were however not changed. We found that the two electrons from O vacancies were ionized and localized on a V and a Bi atom, at the PBE level of theory, as shown in Supplementary Fig. 7 . This makes the charge state of the O vacancy q =+2. Within PBE+ U , the isolated gap states observed within PBE split into two bands, with the spin density mostly localized on V atoms for both states, as shown in Supplementary Fig. 8 . The inclusion of Hubbard U has several effects; it leads to (i) localization of the excess electrons only on V and (ii) an increase in the energy difference between the filled gap states created by oxygen vacancies and the conduction band minimum (mainly composed of V d states) by 0.2 eV, compared with PBE; such differences increase with the magnitude of U , however the charge density remains localized on V atoms for all U values. Small polaron binding energy and mobility The small polaron binding energy ( W p ) can be computed [42] where , ɛ ∞ and ɛ 0 are the high frequency and static dielectric constant respectively; the r p is the small polaron radius. The small polaron radius is on the order of magnitude of 1 Å, and it can be approximately computed as , where is the number of centres per unit volume. The computed ɛ ∞ and ɛ 0 are 6.9 and 52, respectively, for undoped BiVO 4 and we obtain r p =1.73 Å from our DFT calculations (at the PBE level of theory), which gives a polaron binding energy of 0.52 eV. The model adopted here yields a lower bound for the polaron binding energy. The polaron binding energy is non-negligible compared with kT ; hence the formation of small polarons at V sites is energetically favoured. Recent resistivity ( ρ ) measurements [39] on single crystal n-doped BiVO 4 show that between 250 and 400 K, the resistivity data perfectly fit to the adiabatic small polaron model [42] : , where T is the absolute temperature, k is the Boltzmann’s constant and W H is the polaron hopping activation energy. W H may be approximated by , where ɛ p and r p have been defined above [42] , [54] , in the formula giving the polaron binding energy. R is the distance between small polaron hopping centres. We found that ɛ ∞ changed from 6.9 (pristine BiVO 4 ) to 6.2 (doped BiVO 4 with 6% N substitution and 3% O vacancies) and ɛ 0 changed from 52 (pristine BiVO 4 ) to 27 (doped BiVO 4 ). The significant lowering of ɛ 0 stems from the presence of several higher phonon vibrational frequencies present after N-doping ( ɛ 0 is inversely proportional to the square of the phonon vibrational frequencies). Overall, the W H is lowered by 1.1% upon doping, which leads to an improvement in the mobility μ by ∼ 25% according to . DFT calculations for charge-balanced N-doped BiVO 4 Projected density of states of BiVO 4 with charge-balanced N-doping (9% O replaced with 6% N and 3% O vacancy) obtained within DFT-PBE+ U is shown below ( Supplementary Fig. 9 ). In this case, due to the relative proportion of substitutional N atoms and O vacancies, electrons from O vacancies compensate for extra holes generated by N substitution, balancing the charge. For the charge-balanced N-doping, we have also carried out calculations to study the stability of an N dopant and O vacancy complex, by comparing the total energy of a configuration where the O vacancy is far away from a N dopant (at a ∼ 7–10 Å distance) to that of a configuration where the O vacancy is close to a N dopant (at a ∼ 2 Å distance) in which case N dopants and O vacancies interact strongly to form a complex; we used a super cell with two N dopants and one extra O vacancy. We found that the total energy is lowered by 0.26 eV when forming a N dopant–O vacancy complex, which means that the complex defect is thermodynamically preferred; however, the formation of this complex may be kinetically limited, as the N dopant or O vacancy have to migrate towards each other to form the complex. We note that the band structure of the sample where the N dopant–O vacancy complex is present is more dispersive than that where the N dopants and O vacancies are far apart and the bandgap is 0.2 eV higher. DFT calculations for N-doped BiVO 4 with excess oxygen vacancies We performed spin-polarized DFT with the PBE approximation calculations of BiVO 4 with additional O vacancies, in excess to those necessary to charge N-substituted centres (doping concentration of 6% N and 6% O vacancies, see Supplementary Fig. 10 ). As shown in Supplementary Fig. 10 , the N 2 p states lie at the top of valence band and are mixed with O 2 p states; the presence of N leads to an increase of the VBM energy and a decrease of the bandgap of BiVO 4 by 0.3 eV, (The bandgap here is defined as the energy difference between the bottom of the conduction band above the Fermi level and the top of the valence band (mixed O and N 2 p states)). In addition, there are filled gap states due to excess electrons from additional O vacancies, which are localized around V atoms, even with U =0. This is probably due to lattice distortions occurring in the presence of N and favouring localization of electronic states. The major findings in different doping cases are summarized in Supplementary Table 2 . How to cite this article: Kim, T. W. et al . Simultaneous enhancements in photon absorption and charge transport of bismuth vanadate photoanodes for solar water splitting. Nat. Commun. 6:8769 doi: 10.1038/ncomms9769 (2015).